Time-resolved magnetic sensing with electronic spins in diamond Quantum probes can measure time-varying fields with high sensitivity and spatial resolution, enabling the study of biological, material and physical phenomena at the nanometre scale. In particular, nitrogen-vacancy centres in diamond have recently emerged as promising sensors of magnetic and electric fields. Although coherent control techniques have measured the amplitude of constant or oscillating fields, these techniques are not suitable for measuring time-varying fields with unknown dynamics. Here we introduce a coherent acquisition method to accurately reconstruct the temporal profile of time-varying fields using Walsh sequences. These decoupling sequences act as digital filters that efficiently extract spectral coefficients while suppressing decoherence, thus providing improved sensitivity over existing strategies. We experimentally reconstruct the magnetic field radiated by a physical model of a neuron using a single electronic spin in diamond and discuss practical applications. These results will be useful to implement time-resolved magnetic sensing with quantum probes at the nanometre scale. Measurements of weak electric and magnetic fields at the nanometre scale are indispensable in many areas, ranging from materials science to fundamental physics and biomedical science. In many applications, much of the information about the underlying phenomena is contained in the dynamics of the field. While novel quantum probes promise to achieve the required combination of high sensitivity and spatial resolution, their application to efficiently mapping the temporal profile of the field is still a challenge. Quantum estimation techniques [1] , [2] can be used to measure time-varying fields by monitoring the shift in the resonance energy of a qubit sensor, for example, via Ramsey interferometry. The qubit sensor, first prepared in an equal superposition of its eigenstates, accumulates a phase , where γ is the strength of the interaction with the time-varying field b ( t ) during the acquisition period T . The dynamics of the field could be mapped by measuring the quantum phase over successive, increasing acquisition periods [3] or sequential small acquisition steps [4] ; however, these protocols are inefficient at sampling and reconstructing the field, as the former involves a deconvolution problem, while both are limited by short coherence times ( T 2 *) that bound the measurement sensitivity. Decoupling sequences [5] , [6] , [7] could be used to increase the coherence time [8] , [9] , [10] , [11] , but their application would result in a non-trivial encoding of the dynamics of the field onto the phase of the qubit sensor [12] , [13] , [14] , [15] , [16] . Instead, here we propose to reconstruct the temporal profile of time-varying fields by using a set of digital filters, implemented with coherent control sequences over the whole acquisition period T , that simultaneously extract information about the dynamics of the field and protect against dephasing noise. In particular, we use control sequences ( Fig. 1 ) associated with the Walsh functions [17] , which form a complete orthonormal basis of digital filters and are easily implementable experimentally. 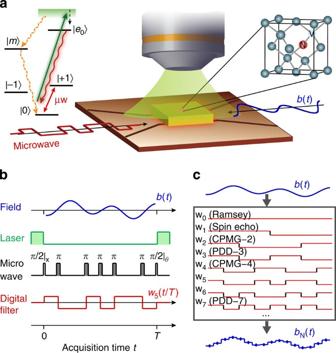Figure 1: Walsh reconstruction protocol. (a) A single nitrogen vacancy centre in diamond, optically initialized and read out by confocal microscopy, is manipulated with coherent control sequences to measure the arbitrary profile of time-varying magnetic fields radiated by a coplanar waveguide under ambient conditions. (b) Coherent control sequences, acting as digital filters on the evolution of the qubit sensor, extract information about time-varying fields. (c) AnN-point functional approximation of the field is obtained by sampling the field with a set ofNdigital filters taken from the Walsh basis, which contain some known set of decoupling sequences such as the even-parity Carr-Purcell-Meiboom-Gill sequences5(w2n) and the odd-parity periodic dynamical decoupling sequences7(w2n-1). Figure 1: Walsh reconstruction protocol. ( a ) A single nitrogen vacancy centre in diamond, optically initialized and read out by confocal microscopy, is manipulated with coherent control sequences to measure the arbitrary profile of time-varying magnetic fields radiated by a coplanar waveguide under ambient conditions. ( b ) Coherent control sequences, acting as digital filters on the evolution of the qubit sensor, extract information about time-varying fields. ( c ) An N -point functional approximation of the field is obtained by sampling the field with a set of N digital filters taken from the Walsh basis, which contain some known set of decoupling sequences such as the even-parity Carr-Purcell-Meiboom-Gill sequences [5] ( w 2 n ) and the odd-parity periodic dynamical decoupling sequences [7] ( w 2 n - 1 ). Full size image The Walsh reconstruction method can be applied to estimate various time-varying parameters via coherent control of any quantum probe. In particular, we show that the phase acquired by a qubit sensor modulated with Walsh decoupling sequences is proportional to the Walsh transform of the field. This simplifies the problem of spectral sampling and reconstruction of time-varying fields by identifying the sequency domain as the natural description for dynamically modulated quantum systems. At the same time, the Walsh reconstruction method provides a solution to the problem of monitoring a time-dependent parameter with a quantum probe, which cannot be in general achieved via continuous tracking due to the destructive nature of quantum measurements. In addition, because the Walsh reconstruction method achieves dynamical decoupling of the quantum probe, it further yields a significant improvement in coherence time and sensitivity over sequential acquisition techniques. These characteristics and the fact that the Walsh reconstruction method can be combined with data compression [18] and compressive sensing [19] , [20] provide clear advantages over prior reconstruction techniques [3] , [4] , [21] , [22] . Walsh reconstruction method The Walsh reconstruction method relies on the Walsh functions ( Supplementary Fig. 1 ), which are a family of piecewise-constant functions taking binary values, constructed from products of square waves, and forming a complete orthonormal basis of digital filters, analogous to the Fourier basis of sine and cosine functions. The Walsh functions are usually described in a variety of labelling conventions, including the sequency ordering that counts the number of sign inversions or ‘switchings’ of each Walsh function. The Walsh sequences are easily implemented experimentally by applying π -pulses at the switching times of the Walsh functions; these sequences are therefore decoupling sequences [23] , [24] , which include the well-known Carr-Purcell-Meiboom-Gill [5] and periodic dynamical decoupling sequences [7] . Because a π -pulse effectively reverses the evolution of the qubit sensor, control sequences of π -pulses act as digital filters that sequentially switch the sign of the evolution between ±1. If w m ( t / T ) is the digital filter created by applying m control π -pulses at the zero crossings of the m -th Walsh function, the normalized phase acquired by the qubit sensor is Here is the m -th Walsh coefficient defined as the Walsh transform of b ( t ) evaluated at sequence number (sequency) m . This identifies the sequency domain as the natural description for digitally modulated quantum systems. Indeed, equation (1) implies a duality between the Walsh transform and the dynamical phase acquired by the qubit sensor under digital modulation, which allows for efficient sampling of time-varying fields in the sequency domain and direct reconstruction in the time domain via linear inversion. Successive measurements with the first N Walsh sequences give a set of N Walsh coefficients that can be used to reconstruct an N -point functional approximation to the field Equation (2) is the inverse Walsh transform of order N , which gives the best least-squares Walsh approximation to b ( t ). With few assumptions or prior knowledge about the dynamics of the field, the reconstruction can be shown to be accurate with quantifiable truncation errors and convergence criteria [25] , [26] . Although the signal is encoded on the phase of a quantum probe in a different way (via decoupling sequences), the Walsh reconstruction method shares similarities with classical Hadamard encoding techniques in data compression, digital signal processing, and nuclear magnetic resonance imaging [27] , [28] , [29] . All of these techniques could easily be combined to achieve both spatial and temporal imaging of magnetic fields at the nanometre scale, given the availability of gradient fields and frequency-selective pulses. Walsh reconstruction of time-varying fields We experimentally demonstrate the Walsh reconstruction method by measuring increasingly complex time-varying magnetic fields. We used a single NV centre in an isotopically purified diamond sample as the qubit sensor (details about the experimental setup can be found in Methods). NV centres in diamond ( Fig. 1a ) have recently emerged as promising sensors for magnetic [30] , [31] , [32] and electric [33] fields, rotations [34] , [35] and temperature [36] , [37] , [38] . These sensors are ideal for nanoscale imaging of living biological systems [39] , [40] , [41] due to their low cytotoxicity, surface functionalizations [42] , optical trapping capability [43] , [44] and long coherence time under ambient conditions [3] . A single NV centre is optically initialized and read out by confocal microscopy under ambient conditions. A coplanar waveguide delivers both resonant microwave pulses and off-resonant time-varying magnetic fields produced by an arbitrary waveform generator. We first reconstructed monochromatic sinusoidal fields, b ( t )= b sin (2 πνt + α ), by measuring the Walsh spectrum up to fourth order ( N =2 4 ). The m -th Walsh coefficient of the normalized field f ( t )= b ( t )/ b was obtained by sweeping the amplitude of the field and measuring the slope of the signal at the origin ( Fig. 2a and Supplementary Fig. 2 ). 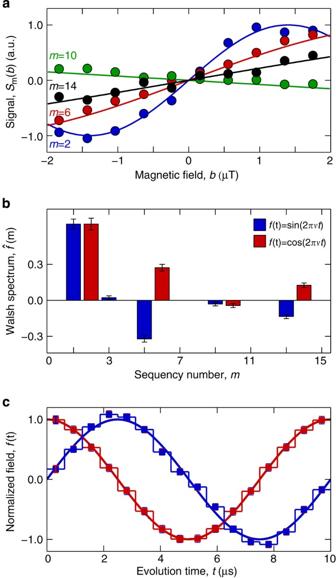Figure 2: Walsh reconstruction of sinusoidal fields. (a) Measured signalas a function of the amplitude of a cosine magnetic field for different Walsh sequences withm π-pulses. Hereγe=2π·28 Hz nT−1is the gyromagnetic ratio of the NV electronic spin. Them-th Walsh coefficientis proportional to the slope ofSm(b) at the origin. (b) Measured Walsh spectrum up to fourth order (N=24) of sine and cosine magnetic fieldsb(t)=bsin (2πνt+α) with frequencyν=100 kHz and phases αε{0,π/2} over an acquisition periodT=1/ν=10 s. Error bars correspond to 95% confidence intervals on the Walsh coefficients associated with the fit of the measured signal. (c) The reconstructed fields (filled squares) are 16-point piecewise-constant approximations to the expected fields (solid lines, not a fit). Error bars correspond to the amplitude uncertainty of the reconstructed field obtained by propagation of the errors on the estimates of the uncorrelated Walsh coefficients. Figure 2b shows the measured non-zero Walsh coefficients of the Walsh spectrum. As shown in Fig. 2c , the 16-point reconstructed fields are in good agreement with the expected fields. We note that, contrary to other methods previously used for a.c. magnetometry, the Walsh reconstruction method is phase selective, as it discriminates between time-varying fields with the same frequency but different phase. Figure 2: Walsh reconstruction of sinusoidal fields. ( a ) Measured signal as a function of the amplitude of a cosine magnetic field for different Walsh sequences with m π -pulses. Here γ e =2 π ·28 Hz nT −1 is the gyromagnetic ratio of the NV electronic spin. The m -th Walsh coefficient is proportional to the slope of S m ( b ) at the origin. ( b ) Measured Walsh spectrum up to fourth order ( N =2 4 ) of sine and cosine magnetic fields b ( t )= b sin (2 πνt +α) with frequency ν =100 kHz and phases αε{0, π /2} over an acquisition period T =1/ ν =10 s. Error bars correspond to 95% confidence intervals on the Walsh coefficients associated with the fit of the measured signal. ( c ) The reconstructed fields (filled squares) are 16-point piecewise-constant approximations to the expected fields (solid lines, not a fit). Error bars correspond to the amplitude uncertainty of the reconstructed field obtained by propagation of the errors on the estimates of the uncorrelated Walsh coefficients. Full size image We further reconstructed a bichromatic field b ( t )= b [ a 1 sin (2 πν 1 t + α 1 )+ a 2 sin (2 πν 2 t + α 2 )]. 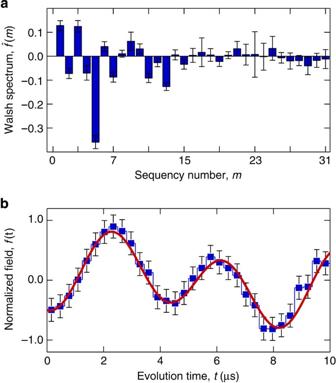Figure 3: Walsh reconstruction of a bichromatic field. (a) Measured Walsh spectrum up to fifth order (N=25) of a bichromatic magnetic fieldb(t)=b[a1sin (2πν1t+α1)+a2sin(2πν2t+α2)] witha1=3/10,a2=1/5,ν1=100 kHz,ν1=250 kHz,α1=−0.0741, andα2=−1.9686. The zero-th Walsh coefficientcorresponds to a static field offset that was neglected. (b) The reconstructed field (filled squares) is a 32-point approximation to the expected field (solid line, not a fit). Error bars correspond to the amplitude uncertainty of the reconstructed field obtained by propagation of the errors on the estimates of the uncorrelated Walsh coefficients. Figure 3a shows the measured Walsh spectrum up to fifth order ( N =2 5 ). As shown in Fig. 3b , the 32-point reconstructed field agrees with the expected field, which demonstrates the accuracy of the Walsh reconstruction method ( Supplementary Fig. 3 ). In contrast, sampling the field with an incomplete set of digital filters, such as the Carr-Purcell-Meiboom-Gill and periodic dynamical decoupling sequences, extracts only partial information about the dynamics of the field ( Supplementary Fig. 4 ). By linearity of the Walsh transform, the Walsh reconstruction method applies to any polychromatic field (and by extension to any time-varying field), whose frequency spectrum lies in the acquisition bandwidth [1/ T , 1/ τ ] set by the coherence time T ≤ T 2 and the maximum sampling time τ = T / N , which is in turn limited by the finite duration of the control π -pulses. Figure 3: Walsh reconstruction of a bichromatic field. ( a ) Measured Walsh spectrum up to fifth order ( N =2 5 ) of a bichromatic magnetic field b ( t )= b [ a 1 sin (2 πν 1 t +α 1 )+ a 2 sin (2 πν 2 t +α 2 )] with a 1 =3/10, a 2 =1/5, ν 1 =100 kHz, ν 1 =250 kHz, α 1 =−0.0741, and α 2 =−1.9686. The zero-th Walsh coefficient corresponds to a static field offset that was neglected. ( b ) The reconstructed field (filled squares) is a 32-point approximation to the expected field (solid line, not a fit). Error bars correspond to the amplitude uncertainty of the reconstructed field obtained by propagation of the errors on the estimates of the uncorrelated Walsh coefficients. Full size image Performance of the Walsh reconstruction method The performance of the Walsh reconstruction method is determined by the reconstruction error e N and the measurement sensitivity η N . The least-squares reconstruction error due to truncation of the Walsh spectrum up to N =2 n coefficients is bounded by e N ≤ (ref. 26 ) and vanishes to zero as N tends to infinity (as needed for perfect reconstruction). This implies that although the resources grow exponentially with n , the error converges exponentially quickly to zero, and only a finite number of coefficients is needed to accurately reconstruct the field. The measurement sensitivity of the m -th Walsh sequence in M measurements, gives the minimum field amplitude, δb m = η m / =Δ S m /(|∂ S m /∂ b m | ), that can be measured with fixed resources. Here γ e =2 π ·28 Hz nT −1 is the gyromagnetic ratio of the NV electronic spin and C accounts for inefficient photon collection and finite contrast due to spin-state mixing during optical measurements [30] , [45] . The sensitivity is further degraded by the decay of the signal visibility, ≤1, where T 2 ( m ) and p ( m ) characterize the decoherence of the qubit sensor during the m -th Walsh sequence in the presence of a specific noise environment. In general, T 2 ( m )> T 2 , as the Walsh sequences suppress dephasing noise and extend coherence times by many orders of magnitude [23] , [24] . The sensitivity η m is thus the ratio between a field-independent factor and the Walsh coefficient for the particular temporal profile of the measured field. The sensitivity formula of equation (3) can be used to identify the Walsh sequences that extract the most information about the amplitude of time-varying fields in the presence of noise. In analogy to a.c. magnetometry [30] , which measures the amplitude of sinusoidal fields, we refer to the problem of performing parameter estimation of the amplitude of an arbitrary waveform as arbitrary waveform (a.w.) magnetometry. Indeed, if the dynamics of the field is known, the Walsh spectrum can be precomputed to identify the Walsh sequence that offers the best sensitivity. Because different Walsh sequences have different noise suppression performances [18] , [23] , the choice of the most sensitive Walsh sequence involves a trade-off between large Walsh coefficients and long coherence times. Measurements with an ensemble of N NV NV centres will improve the sensitivity by 1/ , such that the sensitivity per unit volume will scale as 1/ , where n NV is the density of NV centres. Previous studies have demonstrated η 1 ≈4 nT Hz −1/2 for a single NV centre in an isotopically engineered diamond [3] and η 1 ≈0.1 nT Hz −1/2 for an ensemble of NV centres [46] , with expected improvement down to η 1 ≈0.2 nT μm 3/2 Hz −1/2 . The amplitude resolution of the Walsh reconstruction method, , gives the smallest variation of the reconstructed field that can be measured from the Walsh spectrum of order N . If each Walsh coefficient is obtained from M measurements over the acquisition period N , the measurement sensitivity of the Walsh reconstruction method, η N ≡ δb N , is The Walsh reconstruction method provides a gain in sensitivity of over sequential measurement techniques that perform N successive amplitude measurements over small time intervals of length . Indeed, Walsh sequences exploit the long coherence time under dynamical decoupling to reduce the number of measurements, and thus the associated shot noise. This corresponds to a decrease by a factor of N of the total acquisition time needed to reach the same amplitude resolution or an improvement by a factor of of the amplitude resolution at fixed total acquisition time (see Supplementary Discussion ). Thus, unless the signal can only be triggered once, in which case one should use an ensemble of quantum probes to perform measurements in small time steps, the Walsh reconstruction method outperforms sequential measurements, which is an important step towards quantum-optimized waveform reconstruction [47] . The measurement sensitivity η N combines with the reconstruction error e N to determine the accuracy of the Walsh reconstruction method. If some small coefficients cannot be resolved due to low signal visibility, the increase in reconstruction error can be analytically quantified using data compression results [18] . In the same way, the acquisition time can be reduced by sampling only the most significant coefficients and discarding other negligible coefficients. Furthermore, if the field is sparse in some known basis, which is often the case, a logarithmic scaling in resources can be achieved by using compressed sensing methods based on convex optimization algorithms [19] , [20] , an advantage that is not shared by other sequential acquisition protocols [3] , [4] , [21] . The Walsh reconstruction method is readily applicable to measure time-varying parameters in a variety of physical systems, including light shift spectroscopy with trapped ions [16] ; magnetometry with single spins in semiconductors [31] , [48] , [49] or quantum dots [50] ; and measurements of electric fields [33] or temperature [36] , [37] , [38] with NV centres in diamond. Other promising applications include magnetic resonance spectroscopy of spins extrinsic to the diamond lattice [51] , [52] , measurements of the dynamics of magnetic nanostructures [53] or magnetic vortices in nanodisk chains [54] . An active research direction for quantum sensors is measuring biological [41] , [55] , [56] and neuronal [4] , [57] activity at the nanometre scale. Reference [4] provided compelling evidence about the feasibility of measuring the magnetic fields radiated by action potentials flowing through single neurons. They calculated magnetic field strengths of the order of 10 nT at distance up to 100 nm from a morphologically reconstructed hippocampal CA1 pyramidal neuron. These fields are within experimental reach using small ensembles of shallow-implanted NV centres, for example, located less than 10 nm below the diamond surface [58] , [59] , given improvements in collection efficiency [46] , [60] and coherence times [61] . The Walsh reconstruction method may also prove useful in neuroscience, alongside existing electrical activity recording techniques and other emerging neuroimaging modalities, to monitor the weak magnetic activity of neuronal cells at subcellular spatial resolution, as needed to better understand neurophysiology and map neuronal circuits. To achieve a repeatable signal and reduce stochastic fluctuations during averaging, sequential trains of action potentials could be evoked with conventional electrophysiological techniques, photo-stimulation methods or current injection through underlying nanowire electrode arrays [62] . Technical issues associated with maintaing the stability of the system over long time scale still remain to be solved. As a proof-of-principle experiment, we measured the magnetic field radiated by a physical model of a neuron undergoing an action potential Φ( t ) approximated by a skew normal impulse [63] , [64] , [65] . Due to its linear response in the kHz regime ( Supplementary Fig. 5 ), our coplanar waveguide acts as the physical model of a neuron (see Supplementary Methods ), with the radiated magnetic field given by the derivative of the electric field [66] , [67] : b ( t )= d Φ( t )/ dt ( Supplementary Fig. 6 ). The Walsh coefficients were measured by fixing the amplitude of the field and sweeping the phase of the last read-out pulse to reconstruct the absolute field b ( t ) rather than the normalized field f ( t ). This protocol is in general applicable when the field amplitude is not under experimental control. 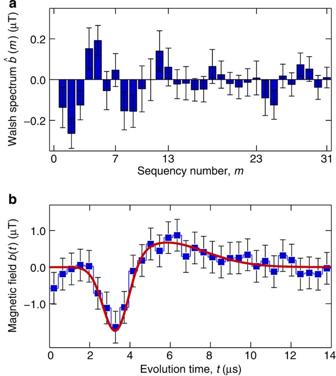Figure 4: Walsh reconstruction of an arbitrary waveform. (a) Measured Walsh spectrum up to fifth order (N=25) of the magnetic field radiated by a skew normal impulse flowing through the physical model of a neuron. The Walsh coefficients were obtained by fixing the amplitude of the field and sweeping the phase of the last read-outπ/2-pulse. The acquisition time for measuring all the Walsh coefficients was less than 4 h. Error bars correspond to 95% confidence intervals on the Walsh coefficients associated with the fit of the measured signal. (b) The reconstructed field (filled squares) is a 32-point approximation to the expected field (solid line, not a fit). Error bars correspond to the amplitude uncertainty of the reconstructed field obtained by propagation of the errors on the estimates of the uncorrelated Walsh coefficients. Figure 4a shows the measured Walsh spectrum up to fifth order ( N =2 5 ). As shown in Fig. 4b , the 32-point reconstructed field is in good agreement with the expected field. Although neuronal fields are typically much smaller than in our proof-of-principle experiment with a single NV centre, they could be measured with shallow-implanted single NVs [51] , [52] , [58] , [59] or small ensembles of NV centres [41] , [46] , [57] . Figure 4: Walsh reconstruction of an arbitrary waveform. ( a ) Measured Walsh spectrum up to fifth order ( N =2 5 ) of the magnetic field radiated by a skew normal impulse flowing through the physical model of a neuron. The Walsh coefficients were obtained by fixing the amplitude of the field and sweeping the phase of the last read-out π /2-pulse. The acquisition time for measuring all the Walsh coefficients was less than 4 h. Error bars correspond to 95% confidence intervals on the Walsh coefficients associated with the fit of the measured signal. ( b ) The reconstructed field (filled squares) is a 32-point approximation to the expected field (solid line, not a fit). Error bars correspond to the amplitude uncertainty of the reconstructed field obtained by propagation of the errors on the estimates of the uncorrelated Walsh coefficients. Full size image In conclusion, we used control sequences acting as digital filters on the evolution of a single NV electronic spin to efficiently sample and accurately reconstruct the arbitrary profile of time-varying fields with quantifiable errors and formal convergence criteria. The Walsh reconstruction method can easily be used together with spatial encoding techniques to achieve both spatial and temporal imaging of magnetic fields. In addition, this method is compatible with data compression techniques [18] and compressed sensing algorithms [19] , [20] to achieve a significant reduction in resources, acquisition time and reconstruction errors. Extension of the Walsh reconstruction method to stochastic fields could simplify the problem of spectral density estimation by removing the need for functional approximations or deconvolution algorithms [13] , [15] , [68] . This would enable, for example, in vivo monitoring of cellular functions associated with cell membrane ion channel processes [55] , [56] . Finally, this work connects with other fields in which the Walsh functions have recently attracted attention, for example, in quantum simulation to construct efficient circuits for diagonal unitaries [69] , in quantum error suppression [23] , [24] , and in quantum control theory to improve the fidelity of two-qubit entangling gates on trapped atomic ions [70] . Nitrogen-vacancy centres in diamond as qubit sensors Measurements of time-varying magnetic fields were performed under ambient conditions with a single NV centre in an isotopically purified diamond sample (>99.99% C-12). The NV centre in diamond consists of a substitutional nitrogen adjacent to a vacancy in the diamond lattice. The negatively charged defect exhibits a ground state electronic spin triplet. The zero-field energy splitting between the m s =0 and m s =±1 sublevels is Δ=2.87 GHz. A static magnetic field b 0 =2.5 mT directed along the quantization axis of the NV centre lifts the energy degeneracy between the m s =+1 and m s =−1 sublevels via the Zeeman effect. This gives an effective spin qubit m s =0↔ m s =1 that can be used to measure time-varying magnetic fields. The strength of the interaction with external magnetic fields is given by the gyromagnetic ratio of the electron γ e =2 π ·28 Hz nT −1 . The NV centre was located in a home-built confocal microscope via fluorescence emission collection and optically initialized to its ground state with a 532 nm laser pulse. Coherent control of the optical ground-state levels of the NV electronic spin was performed with resonant microwave pulses delivered through an on-chip coplanar waveguide. We set the effective Rabi frequency to 25 MHz to achieve 20 ns π -pulses and implemented phase cycling to correct for pulse errors. The coplanar waveguide was also used to deliver non-resonant magnetic fields ( t ) generated with an arbitrary waveform generator. The magnetometry method measured the resonance shift produced by the projection of the time-dependent field along the NV axis, b ( t )= ( t ) z . The qubit was optically read out via spin-state dependent fluorescence measurements in the 600–800 nm spectral window around the 637-nm zero-phonon line with a single-photon counter. Walsh functions The set of Walsh functions [17] , [25] , [26] is a complete, bounded and orthonormal basis of digital functions defined on the unit interval t ε[0,1]. The Walsh basis can be thought of as the digital equivalent of the sine and cosine basis in Fourier analysis. The Walsh functions in the dyadic ordering or Paley ordering are defined as the product of Rademacher functions ( r k ): w 0 =1 and w m = for 1≤ m ≤2 n –1, where m k is the k -th bit of m . The dyadic ordering is particularly useful in the context of data compression [18] . The Rademacher functions are periodic square-wave functions that oscillate between ±1 and exhibit 2 k intervals and 2 k –1 jump discontinuities on the unit interval. Formally, the Rademacher function of order k ≥1 is defined as r k ( t )≡ r (2 k −1 t ), with extended periodically to the unit interval. The Walsh functions in the sequency ordering are obtained from the grey code ordering of m . Sequency is a straightforward generalization of frequency which indicates the number of zero crossings of a given digital function during a fixed time interval. As such, the sequency m indicates the number of control π -pulses to be applied at the zero crossings of the m -th Walsh function. The sequency ordering is thus the most intuitive ordering in the context of digital filtering with control sequences. How to cite this article : Cooper, A. et al. Time-resolved magnetic sensing with electronic spins in diamond. Nat. Commun. 5:3141 doi: 10.1038/ncomms4141 (2014).